Intramolecular charge transfer enables highly-efficient X-ray luminescence in cluster scintillators 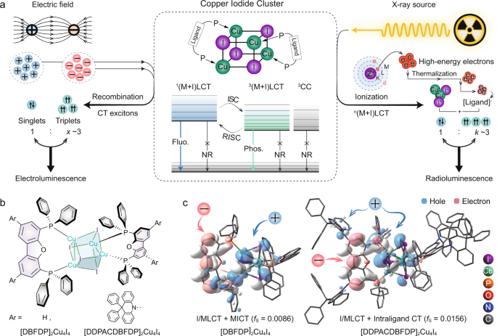Fig. 1: Photo-, electro- and radio-luminescence from Cu4I4cubic scintillators. aEmission mechanisms of Cu4I4cubic clusters. Middle: excited-state composition of Cu4I4cubic clusters stabilized with biphosphine ligands. (M + I)LCT and CC refer to metal and iodide-to-ligand charge transfer and cluster centered metal-to-iodide charge transfer (MICT) excited states, respectively, which induce separated positive and negative charges respectively on Cu4I4cube and peripheral ligands. Superscripts of “1” and “3” denote singlet and triplet states, respectively. Fluorescence, phosphorescence, nonradiation, intersystem crossing and reverse intersystem crossing are abbreviated as Fluo., Phos., NR, ISC and RISC, respectively. Left: in sandwiched light-emitting diode, hole and electron generated by electric field can be captured by Cu4I4cube and ligands to form charge transfer (CT) excitons, corresponding to (M + I)LCT excited states of the clusters, which are then de-excited for electroluminescence (EL). Right: through photoelectric effect and Compton scattering, the inner electrons of Cu and I as heavy atoms are firstly excited by X ray to eject high-energy electrons and ionize Cu4I4cube. The hot electrons further interact with atoms to produce massive secondary electrons. After losing sufficient energy, electrons are finally captured by ligands to form hole-electron pairs. The excited clusters characteristic of (M + I)LCT emit radioluminescence (RL).xandkare ratios of triplet and singlet excitons, and ionized and directly excited molecules, respectively. For both electric field and X-ray excitations, molecular ionization namely (M + I)LCT is dominant, leading toxandkapproaching to three according to spin statistics.bChemical structures of biphosphine stabilized Cu4I4cubes, respectively named [DBFDP]2Cu4I4(Ar = H) and [DDPACDBFDP]2Cu4I4(Ar = 9,9-diphenylacridine, DPAC).cSingle crystal structures of the clusters, whose cubes are highlighted in ball-stick model, and contours of triplet “hole” (blue) and “electron” (pink) for nature transition orbitals (NTO) simulated with time-dependent density functional theory (TDDFT).fSis singlet oscillator strength. Luminescence clusters composed of organic ligands and metals have gained significant interests as scintillators owing to their great potential in high X-ray absorption, customizable radioluminescence, and solution processability at low temperatures. However, X-ray luminescence efficiency in clusters is primarily governed by the competition between radiative states from organic ligands and nonradiative cluster-centered charge transfer. Here we report that a class of Cu 4 I 4 cubes exhibit highly emissive radioluminescence in response to X-ray irradiation through functionalizing biphosphine ligands with acridine. Mechanistic studies show that these clusters can efficiently absorb radiation ionization to generate electron-hole pairs and transfer them to ligands during thermalization for efficient radioluminescence through precise control over intramolecular charge transfer. Our experimental results indicate that copper/iodine-to-ligand and intraligand charge transfer states are predominant in radiative processes. We demonstrate that photoluminescence and electroluminescence quantum efficiencies of the clusters reach 95% and 25.6%, with the assistance of external triplet-to-singlet conversion by a thermally activated delayed fluorescence matrix. We further show the utility of the Cu 4 I 4 scintillators in achieving a lowest X-ray detection limit of 77 nGy s −1 and a high X-ray imaging resolution of 12 line pairs per millimeter. Our study offers insights into universal luminescent mechanism and ligand engineering of cluster scintillators. Solution-processed scintillators have recently received significant attention for their ability to transform X-rays into visible light, making them promising candidates for the development of next-generation, high-performance X-ray detectors in medical imaging and industrial detection [1] , [2] , [3] , [4] . In particular, metal clusters stabilized by organic ligands possess inherent advantages in achieving effective radioluminescence, given that heavy-atom metal elements in the cluster exhibit superior X-ray absorption properties [5] , [6] , [7] , and their associated organic ligands typically exhibit high rates of radiative transition [8] , [9] , [10] , [11] . However, these ligand-capped clusters exhibit both molecular and atomic/ionic electronic characteristics [12] , [13] , [14] , [15] , resulting in complex and volatile emissive behaviors [16] , [17] , [18] , [19] , [20] , [21] . For instance, copper clusters, specifically Cu 4 I 4 cubes [22] , [23] , [24] , are effective in luminescent applications due to their highly rigid cubic structures that suppress John-Teller distortion of excited Cu + ions and reduce structural relaxation-induced energy loss [25] , [26] , [27] , [28] , [29] . Unfortunately, many copper clusters exhibit changeable emissions dependent on stimuli such as pressure [30] , friction [22] , and temperature variation [31] , since they possess multiple charge-transfer excited states, including metal/iodine-to-ligand (M/ILCT) and intramolecular charge-transfer (LCT) states, as well as triplet metal-to-iodine ( 3 MICT) charge-transfer states, also known as cluster-centered ( 3 CC) states [32] . It is noteworthy that the presence of low-energy 3 MICT states can induce multi-channel non-radiative decays, which can significantly impact the luminescent performance of copper clusters [33] , [34] , [35] , [36] . In a typical cluster scintillator, X-rays ionize Cu 4 I 4 to release high-energy electrons that initiate secondary electron cascades through atomic interaction [1] , [37] . These hot electrons quickly become thermalized and are captured by the organic ligands in the cluster scintillator, producing hole-electron pairs that are predominantly characteristic of M/ILCT and LCT states. Under the case of ultraviolet excitation, Cu 4 I 4 cubes exhibit photoluminescence through a process in which larger distinction coefficient organic ligands are primarily excited to generate M/ILCT and LCT states, followed by energy transfer to low-lying MICT states [9] , [38] . The situation of electroluminescence from cluster light-emitting diodes (CLED) is similar to radioluminescence in that ligand-involved charge transfer excited states should still predominate [39] , [40] . Despite electrons mainly being captured by ligands, Cu 4 I 4 with lower ionization potential can directly capture holes, which may increase nonradiative 3 MICT under electric excitation. Hence, we reason that precise control over the intramolecular charge-transfer in Cu 4 I 4 clusters is likely to facilitate efficient radioluminescence through electron and hole transfer from Cu 4 I 4 to ligands while reducing direct excitation and energy transfer to MICT quenching states (Fig. 1a ) [1] , [9] , [37] , [38] . Effective ligand contributions to both “electrons” and “holes” are required at the first singlet (S 1 ) and triplet (T 1 ) states, along with designing coordination rigidity to achieve high molecular rigidity of ligands, minimize structural relaxation-induced energy loss, and enhance X-ray irradiation stability [40] , [41] , [42] . Fig. 1: Photo-, electro- and radio-luminescence from Cu 4 I 4 cubic scintillators. a Emission mechanisms of Cu 4 I 4 cubic clusters. Middle: excited-state composition of Cu 4 I 4 cubic clusters stabilized with biphosphine ligands. (M + I)LCT and CC refer to metal and iodide-to-ligand charge transfer and cluster centered metal-to-iodide charge transfer (MICT) excited states, respectively, which induce separated positive and negative charges respectively on Cu 4 I 4 cube and peripheral ligands. Superscripts of “1” and “3” denote singlet and triplet states, respectively. Fluorescence, phosphorescence, nonradiation, intersystem crossing and reverse intersystem crossing are abbreviated as Fluo., Phos., NR, ISC and RISC, respectively. Left: in sandwiched light-emitting diode, hole and electron generated by electric field can be captured by Cu 4 I 4 cube and ligands to form charge transfer (CT) excitons, corresponding to (M + I)LCT excited states of the clusters, which are then de-excited for electroluminescence (EL). Right: through photoelectric effect and Compton scattering, the inner electrons of Cu and I as heavy atoms are firstly excited by X ray to eject high-energy electrons and ionize Cu 4 I 4 cube. The hot electrons further interact with atoms to produce massive secondary electrons. After losing sufficient energy, electrons are finally captured by ligands to form hole-electron pairs. The excited clusters characteristic of (M + I)LCT emit radioluminescence (RL). x and k are ratios of triplet and singlet excitons, and ionized and directly excited molecules, respectively. For both electric field and X-ray excitations, molecular ionization namely (M + I)LCT is dominant, leading to x and k approaching to three according to spin statistics. b Chemical structures of biphosphine stabilized Cu 4 I 4 cubes, respectively named [DBFDP] 2 Cu 4 I 4 (Ar = H) and [DDPACDBFDP] 2 Cu 4 I 4 (Ar = 9,9-diphenylacridine, DPAC). c Single crystal structures of the clusters, whose cubes are highlighted in ball-stick model, and contours of triplet “hole” (blue) and “electron” (pink) for nature transition orbitals (NTO) simulated with time-dependent density functional theory (TDDFT). f S is singlet oscillator strength. Full size image To validate our hypothesis, we designed [DDPACDBFDP] 2 Cu 4 I 4 (DDPACDBFDP = 10,10'-(4,6-bis(diphenylphosphanyl) dibenzofuran-2,8-diyl)bis(9,9-diphenylacridine)), a cluster with ligands have two rigid, strongly electron-donating 9,9-diphenylacridine (DPAC) groups (Fig. 1b ). Due to the DPAC groups being perpendicular to the dibenzofuran moiety, the lone electron pair of the nitrogen atom in the former is not conjugated with the latter. DPAC donors have little influence on the coordination characteristics of the DBFDP moiety. Single-crystal X-ray diffraction confirmed that [DDPACDBFDP] 2 Cu 4 I 4 preserved a cubic core with nearly unchanged Cu…I and Cu…Cu bond lengths (Fig. 1c and Supplementary Fig. 1 ). In this sense, DPAC donor would enhance ligand-centered charge transfer, but has little influence on X-ray absorption by MICT. To figure out how DPAC donors influence the electronic structure of the cluster, we simulated the ground-state (S 0 ) and transition characteristics of [DBFDP] 2 Cu 4 I 4 and [DDPACDBFDP] 2 Cu 4 I 4 with density functional theory (DFT) (Fig. 1c and Supplementary Fig. 2 ). At S 0 states, both two clusters show similar highest occupied (HOMO) and lowest unoccupied molecular orbitals (LUMO) located on Cu 4 I 4 and dibenzofuran, respectively. Introducing DPAC enhances LCT, therefore deepening the LUMO energy level by 0.33 eV. Consistent with this, the experimentally measured HOMO and LUMO energy levels of [DDPACDBFDP] 2 Cu 4 I 4 are simultaneously deepened by ~0.3 eV, reflecting the significant contributions of its peripheral ligands to charge injection/transfer (Supplementary Fig. 3 and Table S1 ). For the singlet and triplet excitations, “electrons” are centralized on dibenzofuran groups of the clusters. “Holes” of [DBFDP] 2 Cu 4 I 4 are localized on phosphine atoms and Cu 4 I 4 . In contrast, “holes” of [DDPACDBFDP] 2 Cu 4 I 4 partially disperse to DPAC donors. With increased singlet M/ILCT and LCT components, oscillator strength ( f S ) of the S 1 state for [DDPACDBFDP] 2 Cu 4 I 4 is nearly doubled. This rationally mixed S 1 and T 1 states make [DDPACDBFDP] 2 Cu 4 I 4 able to integrate the advantages of MICT in X-ray absorption and M/ILCT and LCT in emission. The electronic absorption spectra of [DDPACDBFDP] 2 Cu 4 I 4 film exhibited mixed charge transfer absorption tails in the range of 350-500 nm (inset of Fig. 2a ), indicating the presence of ligand-to-metal charge transfer (LMCT) and metal-to-ligand charge transfer (MLCT) transitions. Excitation spectra of the two clusters revealed the dominant contribution of ligand-centered charge transfer states to singlet and triplet radiative transitions (Fig. 2a and Supplementary Figs. 4 – 5 ). For [DBFDP] 2 Cu 4 I 4 , its MICT excitation spectrum also included a M/ILCT-attributed band caused by increased ligand-to-Cu 4 I 4 energy transfer. Luminescence of both clusters depended on their respective ligand-centered charge transfer transitions. When doped in traditional BCPO and thermally activated delayed fluorescence (TADF) CzAcSF matrices at a concentration of 20%, the photoluminescence peaks of [DDPACDBFDP] 2 Cu 4 I 4 slightly shift blue by 5–10 nm compared to its neat film (Supplementary Fig. 6 ). However, prompt fluorescence (PF), delayed fluorescence (DF), and phosphorescence (PH) spectra of [DDPACDBFDP] 2 Cu 4 I 4 -based films are comparable at room temperature, indicating near-zero singlet-triplet splitting for effective reverse intersystem crossing (Fig. 2b ). Furthermore, [DDPACDBFDP] 2 Cu 4 I 4 exhibited temperature-independent photoluminescence profiles, indicating its stable excited-state composition (Fig. 2c and Supplementary Figs. 7 – 8 ). In contrast, [DBFDP] 2 Cu 4 I 4 neat film showed that with temperature increasing, its ligand-involved emission bands at ~450 nm slightly enhanced, while the emission intensity of its MICT band at ~550 nm increased and then decreased, indicating a turning point at 230 K due to worsened triplet quenching at high temperature [43] (Supplementary Fig. 7 ). Fig. 2: Optical investigations of [DDPACDBFDP] 2 Cu 4 I 4 -based spin-coated films. a Electronic absorption (blue line) and excitation (yellow line) spectra of neat [DDPACDBFDP] 2 Cu 4 I 4 film. Absorption tail in 400–500 nm is magnified, originated from M/ILCT. b Prompt (PF) and delayed fluorescence (DF) and phosphorescence (PH) spectra of host: x % [DDPACDBFDP] 2 Cu 4 I 4 films recorded in time ranges of <1 µs, 1–200 µs and >200 µs, respectively ( x = 100 for neat film, and 20 for doped films). BCPO is bis-4-((N-carbazolyl)phenyl)phenylphosphine oxide as a high-triplet-energy host, and CzAcSF is 10-(4-((4-(9H-carbazol-9-yl)phenyl)sulfonyl)-phenyl)−9,9-dimethyl-9,10-dihydroacridine as a thermally activated delayed fluorescence (TADF) featured host. c Temperature dependence of steady-state emission spectra for host: x % [DDPACDBFDP] 2 Cu 4 I 4 films. d Temperature dependence of time decays for delayed fluorescence (DF) from host: x % [DDPACDBFDP] 2 Cu 4 I 4 films. Dash arrows mark the variation tendencies along with temperature increasing. e Time-resolved transi e nt emission (TRES) spectra of host: x % [DDPACDBFDP] 2 Cu 4 I 4 films at room temperature. Light blue and yellow dash arrows respectively show the differences regarding to prompt fluorescence (PF) and DF contributions. Insets are time decay curves at peak. Full size image The BCPO matrix effectively suppresses intermolecular interaction-induced quenching (Supplementary Fig. 8b ), leading to an increases in the photoluminescence quantum yield (PLQY, ϕ PL ) from 71% for the neat cluster film to 85% for BCPO:[DDPACDBFDP] 2 Cu 4 I 4 . Further improvement of the PLQY is achieved with the CzAcSF matrix, which provides additional reverse intersystem crossing for triplet-to-singlet conversion, thus reducing triplet concentration quenching and achieving a state-of-the-art ϕ PL of 95% for CzAcSF:[DDPACDBFDP] 2 Cu 4 I 4 . Consistent with this, the decay lifetimes of the doped films (τ 1 = ~ 5.5 µs; τ 2 = ~ 15.0 µs) at room temperature are longer than the neat films (τ 1 = ~ 3.5 µs; τ 2 = ~ 12.0 µs) (Fig. 2d and Supplementary Figs. 9 – 13 ). Furthermore, the CzAcSF-hosted film reveals that decay lifetimes first increase from 20 K to 150 K and then slightly decrease at 150-300 K (Supplementary Fig. 10 ). This is attributed to the complementarily contributed triplet utilization of CzAcSF and the M/ILCT and LCT states of the cluster. In this case, the triplet capture by MICT states of clusters is further limited. Time-resolved emission spectra (TRES) indicate that the BCPO matrix effectively prevents influences of intermolecular interactions on photoluminescence properties of [DDPACDBFDP] 2 Cu 4 I 4 , extending the time range of high photon density (in red and orange colors) to 25 µs (Fig. 2e ). Using the CzAcSF matrix slightly increases time range of high photon density to 30 µs, due to reverse intersystem crossing and Förster energy transfer [44] . In contrast to the MICT-originated PH component of [DBFDP] 2 Cu 4 I 4 neat film, which is directly proportional to temperature (Supplementary Fig. 14 ), TRES profiles of [DDPACDBFDP] 2 Cu 4 I 4 -based films are independent on temperature, reflecting limited MICT components (Supplementary Fig. 15 ). Moreover, CzAcSF matrix stabilizes TRES intensities and contours of the clusters, in contrast to the variability observed with neat and BCPO-hosted films. The predominance of M/ILCT and LCT components is crucial for achieving high luminescence stability and quantum efficiency, which is also in accord to the requirement of X-ray excited emission on highly radiative CT excitons. Therefore, compared to [DBFDP] 2 Cu 4 I 4 , [DDPACDBFDP] 2 Cu 4 I 4 with more efficient M/ILCT and LCT excited components can be superior for radioluminescence applications. To investigate the radioluminescence properties of the clusters, we measured X-ray absorption and emission spectra (Fig. 3 ). The X-ray absorption coefficients of Cu 4 I 4 and P atoms ( Z = 53 and K α = 33.2 keV for iodine; Z = 29 and K α = 9.0 keV for copper; Z = 15 and K α = 2.142 keV for phosphorous) are far greater than those of C, H, N and O atoms ( Z = 1–8, K α = 0.0136–0.531 keV). Furthermore, the high absorbance of the copper-iodine clusters indicates the predominance of their coordination skeletons in X-ray absorption. This is evidenced by not only the identical resonant absorption edges of [DDPACDBFDP] 2 Cu 4 I 4 and [DBFDP] 2 Cu 4 I 4 but also their X-ray absorbance being significantly larger than that of commercial organic scintillator Anthracene (Fig. 3a ). Moreover, we found that the X-ray absorbability of the clusters is directly correlated to the proportions of their coordination skeletons. As a result, the absorption coefficient of [DDPACDBFDP] 2 Cu 4 I 4 , which has larger ligands, is markedly lower than that of [DBFDP] 2 Cu 4 I 4 in X-ray energy range of 1-10 4 keV. However, in the contrast to their X-ray absorbance, we found that the radioluminescence intensity of [DDPACDBFDP] 2 Cu 4 I 4 is 20-fold greater than that of [DBFDP] 2 Cu 4 I 4 . This indicates that the photon conversion efficiency of [DDPACDBFDP] 2 Cu 4 I 4 is significantly higher than that of [DBFDP] 2 Cu 4 I 4 . We also observed that the peak radioluminescence intensity of [DDPACDBFDP] 2 Cu 4 I 4 is even stronger than that of commercial inorganic scintillators cadmium tungstate (CWO) and bismuth germinate (BGO), despite the latter having 1-2 orders of magnitude larger X-ray absorbance (Fig. 3b ). Finally, we calculated that the radioluminescence photon number of [DDPACDBFDP] 2 Cu 4 I 4 is 1.04, 1.77, and 8.69 times greater than those of CWO, BGO, and anthracene, respectively, highlighting its potential to practical applications. Fig. 3: Radioluminescence properties of the Cu 4 I 4 cubic scintillators. a X-ray absorption spectra of [DDPACDBFDP] 2 Cu 4 I 4 , [DBFDP] 2 Cu 4 I 4 and commercial scintillators (cadmium tungstate (CWO), bismuth germinate (BGO) and anthracene) and dependence of radioluminescence spectra for clusters on X-ray tube voltage. b radioluminescence spectra and corresponding total radioluminescence photon numbers of [DDPACDBFDP] 2 Cu 4 I 4 and the commercial scintillators at a dose rate of 278 µGy air s −1 , and comparison on total radioluminescence photon number variation of the clusters at different dose rates. The radioluminescence photon number-dose rate relationship of [DDPACDBFDP] 2 Cu 4 I 4 is linearly fitted. COD refers to coefficient of determination. Detection limit is estimated with 3σ/slope method [47] . c radioluminescence stability of [DDPACDBFDP] 2 Cu 4 I 4 under on-off cycles of X-ray radiation at a dose rate of 278 µGy air s −1 . d Photographs of pure scintillator samples (left), and polydimethylsiloxane (PDMS) hosted [DDPACDBFDP] 2 Cu 4 I 4 film (right) excited by X-ray radiation (X-ray tube voltage, 50 kV; dose rate, 104 µGy air s −1 ). e Schematic of the electronic X-ray imaging by cluster scintillator films. A large-scale PDMS:[DDPACDBFDP] 2 Cu 4 I 4 film serves as the detector placed between a X-ray source and a digital camera. f X-ray image of an integrated circuit board recorded at 50 kV. g High-resolution X-ray image of a gauge for line-pairs per millimeter (LP/mm) enabled by [DDPACDBFDP] 2 Cu 4 I 4 (voltage, 50 kV). Full size image The radioluminescence photon number of [DBFDP] 2 Cu 4 I 4 remained nearly unchanged when the X-ray tube voltage exceeded 30 kV, which is attributed to concentration quenching of its MICT state (Fig. 3a ). In contrast, [DDPACDBFDP] 2 Cu 4 I 4 exhibited continuously increased radioluminescence photons, achieving a 7-fold increase at 50 kV. Importantly, in the range of 0.688–278 µGy S −1 , the radioluminescence photon number of [DDPACDBFDP] 2 Cu 4 I 4 is was indirectly proportional to dose rate (Fig. 3b and Supplementary Figs. 16 − 17 ). Conversely, the increase of radioluminescence photon number for [DDPACDBFDP] 2 Cu 4 I 4 was markedly reduced at dose rates exceeding 139 µGy S −1 , indicating worsened concentration quenching. Consequently, at 278 µGy S −1 , [DDPACDBFDP] 2 Cu 4 I 4 ehibited a luminescence signal ~16 times stronger than [DBFDP] 2 Cu 4 I 4 . Thus, enhanced luminescence from ligand-centered charge transfer states proved to be the key factor inducing largely improved scintillator characteristics of [DDPACDBFDP] 2 Cu 4 I 4 . This results also imlies that exciton formation and allocation follow the charge recombination mechanism after X-ray excitation. Furthermore, the high-intensity X-ray-excited luminescence and linear dependence of photon number on X-ray dose rate led to an low X-ray detection limit of 77 nGy S −1 , which is <2% of the standard X-ray diagnostic dosage of 5.5 µGy S −1, [45] . Even after exposure under 278 µGy S −1 for 20 min, the radioluminescence intensity of [DDPACDBFDP] 2 Cu 4 I 4 remained stable, verifying the high X-ray photostability of cubic Cu 4 I 4 clusters (Fig. 3c ). Additionally, [DDPACDBFDP] 2 Cu 4 I 4 demonstrated good photo- and thermo- stabilities and water tolerance, making it competent for diverse applications in complicated and harsh conditions (Supplementary Fig. 18 ). We further demonstrates the utility of [DDPACDBFDP] 2 Cu 4 I 4 for flexible X-ray radiography by incorporating the cluster scintillators into a polydimethylsiloxane (PDMS) film (Fig. 3d ). This cluster-doped PDMS film was then utilized as a detector placed between an integrated circuit board and a digital camera (Fig. 3e ). Under X-ray excitation, the details of integrated circuit can be visualized (Fig. 3f ). The high resolution of X-ray image was further verified using line pairs per millimeter gauge tests (Fig. 3g ). Even at 12 line pairs per millimeter, the line gap can still be clearly recognized clearly, corresponding to a resolution of <40 μm. To gain further understanding of the impact of ligand-involved charge transfer transitions on charge recombination process, the electroluminescence properties of the clusters were investigated. Owing to the similarity of radioluminescence and electroluminescence mechanisms with respect to hole-electron pair utilization, trilayer CLEDs were fabricated through spin-coating clusters in BCPO and CzAcSF matrices, respectively (Fig. 4a, b and Supplementary Figs. 19 – 21 ). The CzAcSF matrix rendered a 50-fold increase in η EQE for [DBFDP] 2 Cu 4 I 4 , reaching 11.6%, owing to limited MICT. In addition to a state-of-the-art η EQE of 25.6% in CzAcSF matrix, the maximum η EQE of [DDPACDBFDP] 2 Cu 4 I 4 in BCPO matrix (15.1%) was 75-fold of that of [DBFDP] 2 Cu 4 I 4 (0.2%), verifying that the predominance of ligand-centered charge transfer states for the former largely improved exciton radiation (Fig. 4c and Supplementary Figs. 22 – 24 ). It is noteworthy that the maximum internal quantum efficiency (IQE, η IQE ) of CzAcSF:[DDPACDBFDP] 2 Cu 4 I 4 reached 100%, which was consistent with its ϕ PL . On the contrary, BCPO:[DDPACDBFDP] 2 Cu 4 I 4 had the maximum η IQE of ~60%, which was only three quarters of its ϕ PL . This manifests that triplet quenching in BCPO-based devices was more serious than in the corresponding films, due to a larger initial triplet ratio in the devices (75%). Therefore, for radioluminescence process with the same triplet/singlet ratio, the predominance of ligand-centered charge transfer states for [DDPACDBFDP] 2 Cu 4 I 4 gives rise to its markedly improved radioluminescence performance. Fig. 4: Hole-electron-pair coupling for luminescence from Cu 4 I 4 clusters. a Device configuration and energy level structure of spin-coated cluster light-emitting diodes (CLED) and chemical structures of the hosts BCPO and CzAcSF. HOMO and LUMO refer to the highest occupied and the lowest unoccupied molecular orbitals. b Electroluminescence spectra of CLEDs respectively using BCPO (top) and CzAcSF (bottom) as hosts. c Comparison on the maximum external quantum efficiencies of the CLEDs. d Electroluminescence TRES contours (left) of [DDPACDBFDP] 2 Cu 4 I 4 based devices at 50, 100, 200 and 300 K, and emission contours at recombination stage (≤ 20 µs) after applying a 5 V bias pulse at room temperature (right). Arrows show the variation tendencies of DF components. e Comparison on centroid distance (d H - L ), wave function overlap integral (<Ψ H | Ψ L >) and electronic cloud overlap probabilities (<Ψ H 2 | Ψ L 2 >) of the LUMOs and the HOMOs for ground states (S 0 ) and the “hole” and “electron” for the S 1 and T 1 states of the clusters. f Proposed mechanism of enhanced radioluminescence for [DDPACDBFDP] 2 Cu 4 I 4 , in comparison to [DBFDP] 2 Cu 4 I 4 . Full size image We further performed exciton kinetic analysis to further understand the roles of charge transfer transitions on hole-electron pairs (Fig. 4d ). Electroluminescence TRES contours show that electroluminescence lifetimes of BCPO:[DDPACDBFDP] 2 Cu 4 I 4 based devices were shortened at higher temperature (Fig. 4d, left and Supplementary Fig. 24 ), while electroluminescence lifetime variation of CzAcSF:[DDPACDBFDP] 2 Cu 4 I 4 has a turning point at 100 K (Supplementary Fig. 25 ). 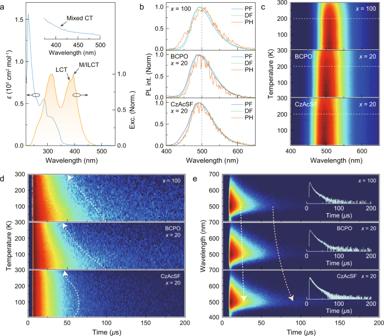Fig. 2: Optical investigations of [DDPACDBFDP]2Cu4I4-based spin-coated films. aElectronic absorption (blue line) and excitation (yellow line) spectra of neat [DDPACDBFDP]2Cu4I4film. Absorption tail in 400–500 nm is magnified, originated from M/ILCT.bPrompt (PF) and delayed fluorescence (DF) and phosphorescence (PH) spectra of host:x% [DDPACDBFDP]2Cu4I4films recorded in time ranges of <1 µs, 1–200 µs and >200 µs, respectively (x= 100 for neat film, and 20 for doped films). BCPO is bis-4-((N-carbazolyl)phenyl)phenylphosphine oxide as a high-triplet-energy host, and CzAcSF is 10-(4-((4-(9H-carbazol-9-yl)phenyl)sulfonyl)-phenyl)−9,9-dimethyl-9,10-dihydroacridine as a thermally activated delayed fluorescence (TADF) featured host.cTemperature dependence of steady-state emission spectra for host:x% [DDPACDBFDP]2Cu4I4films.dTemperature dependence of time decays for delayed fluorescence (DF) from host:x% [DDPACDBFDP]2Cu4I4films. Dash arrows mark the variation tendencies along with temperature increasing.eTime-resolved transient emission (TRES) spectra of host:x% [DDPACDBFDP]2Cu4I4films at room temperature. Light blue and yellow dash arrows respectively show the differences regarding to prompt fluorescence (PF) and DF contributions. Insets are time decay curves at peak. The increased electroluminescence decays at ≥100 K originate from TADF characteristics of CzAcSF, indicating the crucial contribution of CzAcSF matrix to triplet-to-singlet conversion and exciton utilization. We further compared the stages of carrier recombination, energy transfer, and radiation during electroluminescence processes at room temperature (Fig. 4d, right ). Transient emissions from BCPO:[DDPACDBFDP] 2 Cu 4 I 4 based devices corresponded to pure emissions of the cluster, which were time-independent, and started at ~2 µs. On the contrary, in carrier recombination stage, electroluminescence radiation from CzAcSF:[DDPACDBFDP] 2 Cu 4 I 4 was postponed by ~3 µs, which was taken for reverse intersystem crossing by CzAcSF (reverse intersystem crossing rate constant of 8.5 × 10 4 s −1 ) [46] . Furthermore, sky-blue emission from CzAcSF was observed at the beginning. It means excitons were firstly formed on CzAcSF. Then, electroluminescence emission gradually shifted to cluster-originated bluish green (508 nm) at the end of recombination stage and whole decay stage, demonstrating the key advantage of CzAcSF in converging excitons to ligand-centered charge transfer states. Our study shows that the significant increase in the radioluminescence intensity of [DDPACDBFDP] 2 Cu 4 I 4 is coherent with its significantly larger ϕ PL and η EQE . Additionally, MICT-attributed bands in the radioluminescence spectra of [DBFDP] 2 Cu 4 I 4 are considerably stronger than the photoluminescence spectra but comparable to electroluminescence spectra, which implies a similarity between the radioluminescence and electroluminescence mechanisms in exciton formation through charge recombination. To further understand the correlation between the charge transfer characteristics and radioluminescence performance, we compared frontier molecular orbital (FMO) properties of the clusters (Fig. 4e and Supplementary Fig. 26 ). The larger FMO overlaps of the S 0 and S 1 states for [DDPACDBFDP] 2 Cu 4 I 4 favor radiative transition, resulting in stronger radioluminescence emission. Simultaneously, triplet “hole” of [DDPACDBFDP] 2 Cu 4 I 4 is widely distributed on DPAC and partial P…Cu-I moieties apart from the benzofuran-centralized triplet “electrons”. This triplet electronic structure provides an efficient charge-releasing channel from Cu 4 I 4 cube to locally coordinated skeleton during thermalization and generates ligand-involved charge transfer excitons (Fig. 4f ). On the other hand, MICT-predominant triplet state of [DBFDP] 2 Cu 4 I 4 induces the majority of excitons always trapped by its Cu 4 I 4 core. Therefore, high radioluminescence performance of [DDPACDBFDP] 2 Cu 4 I 4 is mainly due to the dominant population of its highly radiative M/ILCT and LCT states. Our study has developed a general ligand-engineering strategy to significantly enhance X-ray luminescent performance of Cu 4 I 4 cubic scintillators through the construction of ligand-centered charge-transfer excited states. Our results demonstrate that the predominance of M/ILCT and LCT states over MICT states is crucial for enhancement of radioluminescence in Cu 4 I 4 clusters. Importantly, the introduction of donor groups in ligands leads to an enhanced emission efficiency by >20-fold for radioluminescence, 14-fold for photoluminescence, and 75-fold for electroluminescence efficiencies in [DDPACDBFDP] 2 Cu 4 I 4 . Moreover, inorganic Cu 4 I 4 and organic ligands complement each other in the radioluminescence process, where the dominance of Cu 4 I 4 in X-ray absorption is overshadowed by the effect of donor groups that induce charge release to the ligand-coordinated skeleton. This leads to the predominance of radiative M/ILCT and LCT states in emission that enables for efficient population of ligand-centered charge-transfer states for high luminescence performance. Our findings offer insights for utilizing organic-inorganic hybrid features of clusters for multiple luminescence applications and benefit the design of high-performance cluster scintillators. Copper iodide cluster synthesis Clusters were synthesized through dissolving 1 mmol of ligand and 2 mmol of CuI in dichloromethane and stirring for several hours to afford crude powder, which was recrystallized to afford white crystals. 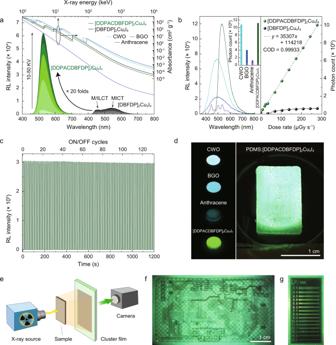Fig. 3: Radioluminescence properties of the Cu4I4cubic scintillators. aX-ray absorption spectra of [DDPACDBFDP]2Cu4I4, [DBFDP]2Cu4I4and commercial scintillators (cadmium tungstate (CWO), bismuth germinate (BGO) and anthracene) and dependence of radioluminescence spectra for clusters on X-ray tube voltage.bradioluminescence spectra and corresponding total radioluminescence photon numbers of [DDPACDBFDP]2Cu4I4and the commercial scintillators at a dose rate of 278 µGyairs−1, and comparison on total radioluminescence photon number variation of the clusters at different dose rates. The radioluminescence photon number-dose rate relationship of [DDPACDBFDP]2Cu4I4is linearly fitted. COD refers to coefficient of determination. Detection limit is estimated with 3σ/slope method47.cradioluminescence stability of [DDPACDBFDP]2Cu4I4under on-off cycles of X-ray radiation at a dose rate of 278 µGyairs−1.dPhotographs of pure scintillator samples (left), and polydimethylsiloxane (PDMS) hosted [DDPACDBFDP]2Cu4I4film (right) excited by X-ray radiation (X-ray tube voltage, 50 kV; dose rate, 104 µGyairs−1).eSchematic of the electronic X-ray imaging by cluster scintillator films. A large-scale PDMS:[DDPACDBFDP]2Cu4I4film serves as the detector placed between a X-ray source and a digital camera.fX-ray image of an integrated circuit board recorded at 50 kV.gHigh-resolution X-ray image of a gauge for line-pairs per millimeter (LP/mm) enabled by [DDPACDBFDP]2Cu4I4(voltage, 50 kV). 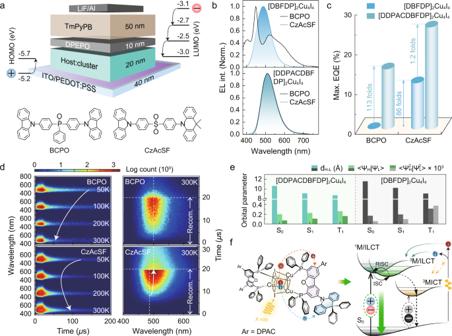Fig. 4: Hole-electron-pair coupling for luminescence from Cu4I4clusters. aDevice configuration and energy level structure of spin-coated cluster light-emitting diodes (CLED) and chemical structures of the hosts BCPO and CzAcSF. HOMO and LUMO refer to the highest occupied and the lowest unoccupied molecular orbitals.bElectroluminescence spectra of CLEDs respectively using BCPO (top) and CzAcSF (bottom) as hosts.cComparison on the maximum external quantum efficiencies of the CLEDs.dElectroluminescence TRES contours (left) of [DDPACDBFDP]2Cu4I4based devices at 50, 100, 200 and 300 K, and emission contours at recombination stage (≤ 20 µs) after applying a 5 V bias pulse at room temperature (right). Arrows show the variation tendencies of DF components.eComparison on centroid distance (dH-L), wave function overlap integral (<ΨH| ΨL>) and electronic cloud overlap probabilities (<ΨH2| ΨL2>) of the LUMOs and the HOMOs for ground states (S0) and the “hole” and “electron” for the S1and T1states of the clusters.fProposed mechanism of enhanced radioluminescence for [DDPACDBFDP]2Cu4I4, in comparison to [DBFDP]2Cu4I4. Detailed experimental procedures are provided in the Supplementary Information. Radioluminescence analysis An X-ray detector was put on film surface. A beam of X-ray source (P357, VJ Technologies) was applied to the electronic board with different amounts of X-ray exposure. Spectra and images were recorded using a spectrometer and an optical microscope, respectively. Additional measurement details are provided in the Supplementary Information. Photoluminescence spectroscopy analysis Steady-state and transient emission measurements were performed using an Edinburgh FLS 1000 fluorescence spectrophotometer equipped with Xenon lamp for 200–900 nm measurement, nano- and microsecond pulsed lamps for 100 ps-10s measurement and a temperature controller for 11-500 K measurement. Electroluminescence analysis The devices were fabricated through spin-coating for emissive layers and vacuum evaporation for electron-transporting layers and cathodes, respectively. A system composed of a Keithley 4200 source meter, a calibrated silicon photodiode and a PR655 spectrum colorimeter was used to measure voltage-current density-luminance characteristics and electroluminescence spectra. Transient and temperature-dependent electroluminescence spectral measurements were performed with FLS 1000 by incorporating a Tektronix AFG3022G function generator.